Intracellular CD24 disrupts the ARF–NPM interaction and enables mutational and viral oncogene-mediated p53 inactivation CD24 is overexpressed in nearly 70% human cancers, whereas TP53 is the most frequently mutated tumour-suppressor gene that functions in a context-dependent manner. Here we show that both targeted mutation and short hairpin RNA (shRNA) silencing of CD24 retard the growth, progression and metastasis of prostate cancer. CD24 competitively inhibits ARF binding to NPM, resulting in decreased ARF, increase MDM2 and decrease levels of p53 and the p53 target p21/CDKN1A . CD24 silencing prevents functional inactivation of p53 by both somatic mutation and viral oncogenes, including the SV40 large T antigen and human papilloma virus 16 E6-antigen. In support of the functional interaction between CD24 and p53, in silico analyses reveal that TP53 mutates at a higher rate among glioma and prostate cancer samples with higher CD24 mRNA levels. These data provide a general mechanism for functional inactivation of ARF and reveal an important cellular context for genetic and viral inactivation of TP53 . CD24 is a glycosyl-phosphatidyl-inositol (GPI)-anchored cell surface molecule. Although found in many tissues, CD24 is most abundant in haematopoietic and immature neuronal cells [1] . Accumulating data have demonstrated that CD24 is among the most overexpressed protein in cancer cells [2] and is a valuable marker indicative of poor prognosis for cancer patients, such as those with non-small-cell lung cancer [3] , colon cancer [4] , oesophageal squamous cell carcinoma [5] , hepatocellular carcinoma [6] , ovarian [7] , breast [8] , glioma [9] , [10] and prostate [11] cancers. The role of CD24 in tumour cell growth has been demonstrated by ectopic and/or inducible expression [12] , [13] , targeted mutation [14] , gene silencing [12] and antibody blocking [15] . By localizing to caveolae, CD24 associates with Src family members, such as Src, Lck and Lyn [16] , [17] , [18] , [19] , linking CD24 to activation of intracellular signal transduction cascades. In addition, cell surface CD24 is often implicated in tumour metastasis [19] , [20] , [21] , [22] , [23] , as fucosylated CD24 interacts with P- and E-selectin, mediating rolling along the endothelium and allowing invasion of tumour cells to distal sites [24] , [25] , [26] . Biogenesis of cell surface proteins involves elongation arrest caused by interaction of the signal peptide with the signal recognition protein. This pause occurs normally when the nascent chain reaches an average of 70 amino acids [27] . As CD24 has an open-reading frame of 76 or 80 amino acids in mouse and human, respectively [28] , [29] , translation of CD24 may have occurred before translocation to the endoplasmic reticulum. Thus, unless degraded, a significant population of CD24 may reside intracellularly, by default. In addition, intracellular CD24 may accumulate in cancer samples because of widespread disruption of genes involved in the processing of GPI-anchored molecules [30] . For example, in colon cancer, intracellular CD24 is associated with cancer prognosis [4] . The significance and mechanism of intracellular CD24 in tumour progression has not been studied. The p19Arf(p14ARF)/p16INK4a locus is unique in cancer biology as it encodes two potential tumour-suppressor genes by using different open-reading frames and a distinct exon 1 (ref. 31 ). ARF and p16 act through the p53 and Rb pathways, respectively [32] , [33] , [34] , [35] . ARF promotes p53 function by inactivating MDM2 (ref. 33 ), the E3 ligase that ubiquitinates p53 and targets it for degradation [36] . The significance of the individual gene products in human tumorigenesis is unclear as selective genetic inactivation of either ARF or INK4a is rare in human cancer samples [37] . Given the strong cancer phenotype in mice with selective inactivation of Arf (ref. 32 ), it is surprising that genetic inactivation of p14ARF alone rarely occurs in human cancer [37] . The scarcity of mutations in p14ARF has roused scepticism of the significance of ARF as a tumour suppressor [37] . However, it is also possible that other mechanisms are responsible for ARF inactivation. In this context, it is of note that the nucleolar protein NPM/B23 interacts with ARF and protects it from degradation [38] . TP53 is the most frequently mutated tumour-suppressor gene [39] . Unlike APC , another frequently mutated tumour suppressor in intestinal cancer [40] , most TP53 mutations are missense and thus allow production of full-length mutant p53 proteins [39] . Perhaps due to reduced expression of the p53 target gene MDM2 , mutant p53 often accumulates at higher levels [41] . Although most TP53 mutations are presumed loss-of-function, some p53 mutants have oncogenic function [42] , [43] , whereas others exhibit a temperature-sensitive phenotype [44] . Understanding the cellular context of p53 mutant function may help restore its tumour-suppressor function while disabling its oncogenic activity. Here we provide a missing link between CD24 overexpression and functional inactivation of the tumour-suppressor genes TP53 and ARF . Cd24 deletion retards development of prostate cancer To test Cd24 function in a spontaneous cancer model, we crossed the Cd24 -null allele [45] into TRAMP mice, a transgenic model that develops spontaneous prostate adenocarcinoma due to the expression of the SV40 T antigen under control of the rat probasin promoter [46] . As shown in Fig. 1a , the onset of palpable tumour development in the prostate of TRAMP mice was significantly delayed by deletion of either one or two alleles of the Cd24 gene. When the prostate size was measured at 30 weeks by magnetic resonance imaging (MRI), the prostate volume was significantly reduced in a gene dose-dependent manner ( P =0.0026, analysis of variance trend test; Fig. 1b,c ). At 35 weeks, the mice were killed and their prostates were weighted. CD24 deficiency also decreased the prostate weight at 35 weeks ( Fig. 1d ). As shown in Fig. 1e and Supplementary Fig. 1 and summarized in Fig. 1f , the majority of cancer in wild-type (WT) TRAMP mice had progressed to poorly differentiated adenocarcinomas (7/12) and distal metastases (8/12) into the kidneys, lungs and liver. In contrast, only 1 mouse in the Cd24 −/− (1/9) and Cd24 +/− (1/12) cohorts developed poorly differentiated adenocarcinomas, whereas 1/12 Cd24 +/− and 0/9 Cd24 −/− mice had metastasis. Therefore, in addition to reduced tumour size, inactivation of a single allele of Cd24 significantly reduced the malignancy of the tumours. 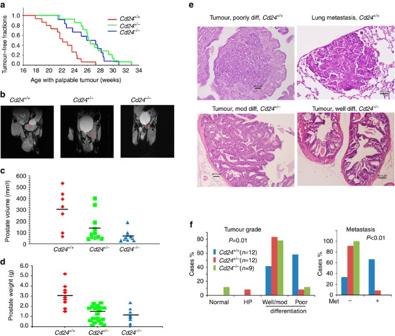Figure 1:Cd24promotes onset and progression of prostate cancer in TRAMP mice. (a) Onset of palpable prostate tumour development inCd24+/+, Cd24+/−andCd24−/−TRAMP mice was observed over 35 weeks.P-value of log-rank tests areCd24WT versusCd24+/−,P=0.0001;Cd24WT versusCd24−/−,P=0.0017;Cd24+/−versusCd24−/−,P=0.51. (b) Representative images of prostates from 30-week-oldCd24+/+(n=7), Cd24+/−(n=11) andCd24−/−(n=9) TRAMP mice. (c) Prostate sizes in 30-week-old TRAMP mice inCd24+/+, Cd24+/−andCd24−/−TRAMP mice. The lower abdominal area was divided into 0.4-mm-thick slices and MRI images were acquired to provide continuous images of the whole prostate. The surface area of the prostate slices was traced by segmenting and summed to estimate the total volume. Analysis of variance (ANOVA) tests revealed an extremely significantCd24gene dose effect on the prostate size (P=0.00026). (d) The weights of 35-week-oldCd24+/+(n=9),Cd24+/−(n=22) andCd24−/−(n=10) TRAMP prostates. ANOVA tests revealed an extremely significant Cd24 gene-dose effect on the prostate weight (P=0.00011). (e) Representative histology of prostate carcinomas (PCa) that developed inCd24+/+Cd24+/−, andCd24−/−TRAMP mice. The data show a difference in the degree of differentiation in tumour morphology. (f) Cd24 promotes progression (left panel) and metastasis (right panel) of prostate cancer in the TRAMP model. The prostate tissue was examined double blind and classified into the following categories: normal prostate, hyperplasia prostate (HP), intraepithelial neoplasia in the prostate (PIN), moderate (mod) to well-differentiated (well diff) PCa and poorly differentiated PCa. Cancer was scored metastatic if one or more distal metastases to either the lungs, kidneys or liver were detected histologically. Examples of tumours at each grade are shown ine, whereas that of normal prostate and hyperplasia are shown inSupplementary Fig. 1. Pearson’sχ2test was used to determine whether theCd24geneotypes affected the progression to poorly differentiated PCa (left panel) or distal metastasis (right panel). Figure 1: Cd24 promotes onset and progression of prostate cancer in TRAMP mice. ( a ) Onset of palpable prostate tumour development in Cd24 +/+ , Cd24 +/− and Cd24 −/− TRAMP mice was observed over 35 weeks. P -value of log-rank tests are Cd24 WT versus Cd24 +/− , P =0.0001; Cd24 WT versus Cd24 −/− , P =0.0017; Cd24 +/− versus Cd24 −/− , P =0.51. ( b ) Representative images of prostates from 30-week-old Cd24 +/+ ( n =7) , Cd24 +/− ( n =11) and Cd24 −/− ( n =9) TRAMP mice. ( c ) Prostate sizes in 30-week-old TRAMP mice in Cd24 +/+ , Cd24 +/− and Cd24 −/− TRAMP mice. The lower abdominal area was divided into 0.4-mm-thick slices and MRI images were acquired to provide continuous images of the whole prostate. The surface area of the prostate slices was traced by segmenting and summed to estimate the total volume. Analysis of variance (ANOVA) tests revealed an extremely significant Cd24 gene dose effect on the prostate size ( P =0.00026). ( d ) The weights of 35-week-old Cd24 +/+ ( n =9), Cd24 +/− ( n =22) and Cd24 −/− ( n =10) TRAMP prostates. ANOVA tests revealed an extremely significant Cd24 gene-dose effect on the prostate weight ( P =0.00011). ( e ) Representative histology of prostate carcinomas (PCa) that developed in Cd24 +/+ Cd24 +/− , and Cd24 −/− TRAMP mice. The data show a difference in the degree of differentiation in tumour morphology. ( f ) Cd24 promotes progression (left panel) and metastasis (right panel) of prostate cancer in the TRAMP model. The prostate tissue was examined double blind and classified into the following categories: normal prostate, hyperplasia prostate (HP), intraepithelial neoplasia in the prostate (PIN), moderate (mod) to well-differentiated (well diff) PCa and poorly differentiated PCa. Cancer was scored metastatic if one or more distal metastases to either the lungs, kidneys or liver were detected histologically. Examples of tumours at each grade are shown in e , whereas that of normal prostate and hyperplasia are shown in Supplementary Fig. 1 . Pearson’s χ 2 test was used to determine whether the Cd24 geneotypes affected the progression to poorly differentiated PCa (left panel) or distal metastasis (right panel). Full size image Cd24-deficient mice have a normal prostate morphology ( Supplementary Fig. 2 ) with comparable numbers of luminal and basal epithelial cells ( Supplementary Fig. 3a ) and prostate weights ( Supplementary Fig. 3b ). In addition, SV40 T antigen was expressed in both normal and malignant cells of the CD24-deficient prostate in TRAMP mice ( Supplementary Fig. 4a ), consistent with normal expression of probasin ( Supplementary Fig. 4b ), the promoter used to drive expression of SV40 T antigen. These data suggest that the reduction in prostate cancer incidence was not due to a lack of SV40-expressing cells. Probing Oncomine.com database revealed that CD24 mRNA is overexpressed in prostate cancer tissues ( Fig. 2a ). In the TRAMP model, Cd24 was expressed in cancer cells but not in the normal prostate gland ( Fig. 2b ). Heterozygous deletion of Cd24 resulted in a quantitative reduction of Cd24 protein ( Fig. 2c ). As Cd24 is highly expressed in haematopoietic cells and plays important roles in both adaptive and innate immunity, we sought to determine whether the Cd24 status in the haematopoietic cells contributes to tumorigenicity. To achieve this goal, we lethally irradiated Cd24 +/+ TRAMP mice and transplanted them with bone marrow from either Cd24 −/− or Cd24 +/+ mice ( Fig. 2d ). Tumour development in the prostate was measured by MRI at 30 weeks and confirmed by histology. In the chimera mice, all leukocytes expressed Cd24 according to the genotype of donor cells ( Fig. 2e ), confirming complete replacement of the haematopoietic system. However, in two independent experiments, the genotype of bone marrow-derived cells had no impact on prostate size ( Fig. 2f ). Thus, prostate tumorigenesis was independent of Cd24 status in the haematopoietic cells. 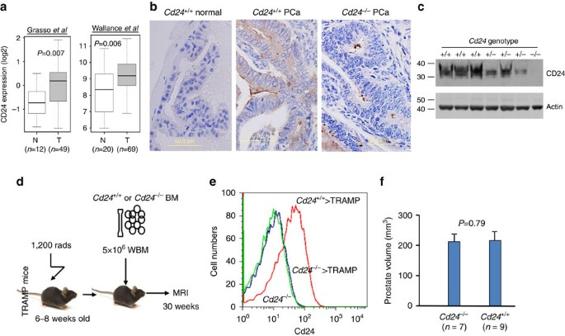Figure 2: Cd24 in non-haematopoietic cells contributes to tumour growth. (a) Overexpression ofCD24mRNA in human prostate cancer tissue based on analysis of two data cohort deposited in Oncomine.com. Two reported cohorts with a sufficient number of matched cancer and normal tissue were analysed.P-values were calculated by Student’st-tests69,70. (b) Expression of Cd24 inCd24+/+PCa but notCd24−/−PCa or normalCd24+/+prostate epithelia. Data shown are representative images and have been reproduced three times. (c) Cd24 levels in TRAMP prostate are gene-dose dependent. Age-matchedCd24+/+andCd24+/−prostate were analysed for Cd24 levels by western blot. (d) Diagram of experimental design. Eight-week-oldCd24+/+TRAMP mice were lethally irradiated and transplanted with 5 × 106bone marrow cells at 1 day after irradiation. The prostate size was measured by MRI at 30 weeks of age. (e) Successful replacement of haematopoietic cells from the donor bone marrow based on Cd24 expression. (f) Means and s.d. of the prostate volume in the bone marrow chimera mice. Figure 2: Cd24 in non-haematopoietic cells contributes to tumour growth. ( a ) Overexpression of CD24 mRNA in human prostate cancer tissue based on analysis of two data cohort deposited in Oncomine.com. Two reported cohorts with a sufficient number of matched cancer and normal tissue were analysed. P -values were calculated by Student’s t -tests [69] , [70] . ( b ) Expression of Cd24 in Cd24 +/+ PCa but not Cd24 −/− PCa or normal Cd24 +/+ prostate epithelia. Data shown are representative images and have been reproduced three times. ( c ) Cd24 levels in TRAMP prostate are gene-dose dependent. Age-matched Cd24 +/+ and Cd24 +/− prostate were analysed for Cd24 levels by western blot. ( d ) Diagram of experimental design. Eight-week-old Cd24 +/+ TRAMP mice were lethally irradiated and transplanted with 5 × 10 6 bone marrow cells at 1 day after irradiation. The prostate size was measured by MRI at 30 weeks of age. ( e ) Successful replacement of haematopoietic cells from the donor bone marrow based on Cd24 expression. ( f ) Means and s.d. of the prostate volume in the bone marrow chimera mice. Full size image Intracellular CD24 promotes growth of cancer cells As the first step to assess the function of CD24 in the growth of human prostate cancer cell lines, we analysed the expression of CD24 mRNA and protein from three cell lines, DU145, LNCaP and PC3. As shown in Fig. 3a , DU145 expressed the highest levels of CD24 mRNA, whereas LNCaP did not express detectable levels. A moderate level of CD24 mRNA was observed in the PC3 cell line. To determine the function of CD24 in DU145 proliferation, we used two independent shRNAs to silence CD24 expression. As shown in Fig. 3b,c , both shRNAs reduced CD24 mRNA levels by approximately fourfold and CD24 protein levels to barely detectable levels. In both 3-(4,5-dimethylthiazol-2-yl) 2,5-diphenyltetrazolium bromide ( Fig. 3d ) and colony formation ( Fig. 3e ) assays, a significant reduction in DU145 growth was observed after silencing CD24. Consistent with this observation, the growth rates of the DU145 tumour in immunodeficient Il2Rg −/− Nod.Scid (NSG) mice ( Fig. 3f ) and nu/nu mice ( Supplementary Fig. 5 ) were substantially reduced ( Fig. 3f ). The role for CD24 in tumour growth is further substantiated by a significant reduction in terminal tumour weight ( Fig. 3g ). 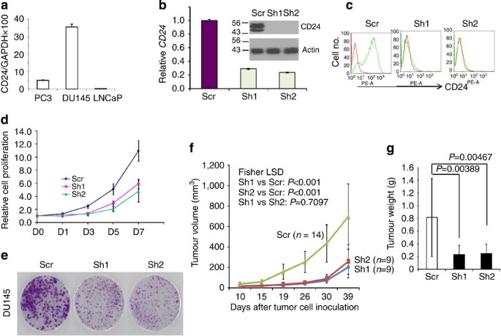Figure 3: CD24 promotes growth of DU145 cells. (a)CD24mRNA levels in three human prostate cancer cell lines are displaced as % of glyceraldehyde 3-phosphate dehydrogenase (GAPDH). (b) Efficient gene silencing of the CD24 gene based on the protein (insert, representative images that have been reproduced three times) and RNA levels. (c) ShRNA silencing eliminates cell surface CD24 expression as determined by flow cytometry. Data shown are representative profiles and have been reproduced three times. (d) ShRNA silencing of CD24 reduces the growth rate as measured by the 3-(4,5-dimethylthiazol-2-yl) 2,5-diphenyltetrazolium bromide assay. Means and s.d. of the relative cell proliferation are shown on the given days. The study has been reproduced three times. (e) Reduced growth rate of tumour cells based on colony size. Data shown are representative images and have been reproduced three times. (f) ShRNA silencing of CD24 reduced the tumour growth in theIl2rg−/−NOD.SCID(NSG) mice. The mice received a subcutaneous injection of 5 × 106tumour cells. Data shown are means and s.d. of the tumour volumes. (g) Weights of tumours at day 39. Error bars, s.d. Scrn=14, Sh1,n=9, Sh2n=9 forfandg. Substantially similar data were obtained when the cells were injected into nu/nu mice. Figure 3: CD24 promotes growth of DU145 cells. ( a ) CD24 mRNA levels in three human prostate cancer cell lines are displaced as % of glyceraldehyde 3-phosphate dehydrogenase (GAPDH). ( b ) Efficient gene silencing of the CD24 gene based on the protein (insert, representative images that have been reproduced three times) and RNA levels. ( c ) ShRNA silencing eliminates cell surface CD24 expression as determined by flow cytometry. Data shown are representative profiles and have been reproduced three times. ( d ) ShRNA silencing of CD24 reduces the growth rate as measured by the 3-(4,5-dimethylthiazol-2-yl) 2,5-diphenyltetrazolium bromide assay. Means and s.d. of the relative cell proliferation are shown on the given days. The study has been reproduced three times. ( e ) Reduced growth rate of tumour cells based on colony size. Data shown are representative images and have been reproduced three times. ( f ) ShRNA silencing of CD24 reduced the tumour growth in the Il2rg −/− NOD.SCID (NSG) mice. The mice received a subcutaneous injection of 5 × 10 6 tumour cells. Data shown are means and s.d. of the tumour volumes. ( g ) Weights of tumours at day 39. Error bars, s.d. Scr n =14, Sh1, n =9, Sh2 n =9 for f and g . Substantially similar data were obtained when the cells were injected into nu/nu mice. Full size image To understand the molecular mechanism by which CD24 silencing causes growth suppression, we compared the gene expression profiles of scrambled, non-silenced control (Scr) versus CD24 shRNA-silenced DU145 cells by gene array analysis. Using P <0.001 and less than 66% or greater than 150% of control levels as a cutoff, we found that as a result of CD24 gene silencing, 408 genes were downregulated, whereas 618 genes were upregulated ( Fig. 4a and Supplementary Data set 1 ). The top ten pathways affected are listed in Supplementary Table 1 . Among them, the most significantly affected pathway was cell cycle regulation ( P =2 × 10 − 5 ). For example, the CDKN1A mRNA, which encodes p21, was significantly elevated ( Fig. 4b ). This increase in p21 corresponded with elevated levels of p53 protein ( Fig. 4c ). Given the function of p21/CDKN1A in G1 arrest, we evaluated the role of CD24 in cell entry into S phase and beyond. We starved DU145 cells under serum-free conditions for 48 h, which arrested the cells at the G0-G1 phase. After 24 h of serum stimulation, more than 70% of the scrambled shRNA-transduced DU145 cells were at either S or G2-M phases ( Fig. 4d ). In contrast, only 39–49% of the CD24 shRNA-transduced cells entered S or G2-M phases ( Fig. 4d ). Therefore, CD24 contributes to cell re-entry into cell cycle following starvation. To determine whether CD24 overexpression is sufficient to promote tumour cell growth, we ectopically expressed CD24 in the LNCaP cell line that does not express CD24. As shown in Fig. 4e , CD24 expression reduced p53 and p21 without marked effect on p27. Consistent with reduced expression of tumour-suppressor genes, CD24 increased LNCaP cell proliferation ( Fig. 4f ). 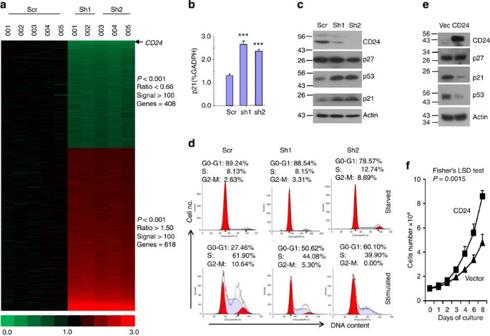Figure 4: CD24 reduces levels of p53 and p21 and promotes tumour cell proliferation. (a) Heat-map depiction of alterations in gene expression in DU145 cells following CD24 gene silencing. RNA isolated from five independent cultures of Scr, three cultures of Sh1 and three cultures of Sh2 were compared using Affymeatrix Human U133 Plus 2.0 microarrays. Only those genes that met the statistical threshold ofP<0.001 and mean alterations that reached the cutoff of >150% or<66% of Scr levels are displayed. The genes are listed inSupplementary Data setand the pathway analysis summary of affected genes is provided inSupplementary Table 1. (b) CD24 silencing increasesp21/CDKN1AmRNA. Error bars, s.d.n=3. The data have been reproduced three times. (c)CD24silencing increased levels of p53 and p21 proteins, but not p27 protein. Representative images of western blots are shown and the data have been reproduced three times. (d) CD24 silencing reduces cell cycle re-entry after starvation. Scr, Sh1 and Sh2 clones were starved for 48 h in serum-free medium and then shifted into serum containing medium. The cells were harvested and analysed for cell cycle progression based on DNA content. These data have been reproduced three times. (e) Ectopic expression of CD24 in LNCaP cell line decreases levels of p53 and p21, but not p27. Representative images of western blots are shown and the data have been reproduced two times. (f) CD24 transduction increases proliferation of LNCaP cells. Data shown are triplicate means and s.d. of triplicates and have been reproduced twice. LSD, least significant difference. Figure 4: CD24 reduces levels of p53 and p21 and promotes tumour cell proliferation. ( a ) Heat-map depiction of alterations in gene expression in DU145 cells following CD24 gene silencing. RNA isolated from five independent cultures of Scr, three cultures of Sh1 and three cultures of Sh2 were compared using Affymeatrix Human U133 Plus 2.0 microarrays. Only those genes that met the statistical threshold of P <0.001 and mean alterations that reached the cutoff of >150% or<66% of Scr levels are displayed. The genes are listed in Supplementary Data set and the pathway analysis summary of affected genes is provided in Supplementary Table 1 . ( b ) CD24 silencing increases p21/CDKN1A mRNA. Error bars, s.d. n =3. The data have been reproduced three times. ( c ) CD24 silencing increased levels of p53 and p21 proteins, but not p27 protein. Representative images of western blots are shown and the data have been reproduced three times. ( d ) CD24 silencing reduces cell cycle re-entry after starvation. Scr, Sh1 and Sh2 clones were starved for 48 h in serum-free medium and then shifted into serum containing medium. The cells were harvested and analysed for cell cycle progression based on DNA content. These data have been reproduced three times. ( e ) Ectopic expression of CD24 in LNCaP cell line decreases levels of p53 and p21, but not p27. Representative images of western blots are shown and the data have been reproduced two times. ( f ) CD24 transduction increases proliferation of LNCaP cells. Data shown are triplicate means and s.d. of triplicates and have been reproduced twice. LSD, least significant difference. Full size image Interestingly, cell surface staining by flow cytometry revealed that only DU145 cells expressed cell surface CD24 ( Fig. 5a ). To determine whether CD24 is expressed intracellularly, we fixed the cells with 4% paraformaldehyde and permeabilized them with detergent to allow antibody access to intracellular CD24. As shown in Fig. 5a , permeabilization increased the levels of CD24 detected in a cell by an average of fivefold in DU145 cells. Thus, the majority of CD24 must reside intracellularly. To determine whether CD24 resides in the cytoplasm or in the nucleus, we compared the amount of CD24 in 0.1% NP-40 soluble (cytoplasmic and plasma membrane) and insoluble (putatively nuclear) fractions. The 0.1% NP-40 insoluble fraction was incubated in 3 mM EDTA and 0.2 mM EGTA to isolate the nucleoplasm. CD24 was detected in both cytoplasmic and nuclear fractions ( Fig. 5b ). As membrane-bound GPI-anchored molecules may be insoluble because of its association with caveolae [47] , we used confocal microscopy to confirm the intracellular distribution of CD24 relative to that of microtubules and DNA. We observed increased CD24 levels and alterations in CD24 distribution during mitosis. As shown in Fig. 5c and Supplementary Fig. 6 , compared with interphase, increased levels of CD24 were found in prophase and metaphase. Also during metaphase, CD24 seemed to distribute itself more evenly with less staining of CD24 in the membrane and more staining in the cytoplasm. This shift was reversed as the cells entered telophase. To confirm the increase in CD24 levels, we arrested DU145 cells at G2 using nocodazole and assessed CD24 protein levels at different time points following nocodazole removal. Concomitant with an increase in Cyclin B1, a marked increase of CD24 was observed as early as 30 min after removal of nocodazole. The increase was transient and largely disappeared at 2 h after nocodazole removal ( Fig. 5d ). 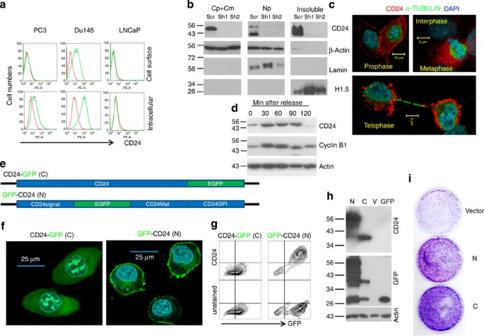Figure 5: Intracellular CD24 and proliferation of prostate cancer cells. (a) Measurement of cell surface and total cellular CD24 by flow cytometry. The prostate cancer cell lines PC3, DU145 and LNCaP were stained with anti-CD24 with or without permeabilization to measure either cell surface (top) or total cellular CD24 (bottom). (b) Analysis of CD24 in the cytoplasmic and plasma membrane fraction (Cp+Cm), nucleoplasm (Np) and the insoluble fraction that includes chromatin by western blot. The efficiency of the fractionation was monitored by the presence of β-actin (Cp+Cm+Np), Lamin (Np) and H1.5 (chromatin). (c) Confocal microscopy reveals dynamic upregulation and localization of CD24 during mitosis. Note alterations of CD24 distribution and signal intensity at different phases during mitosis. SeeSupplementary Fig. 6for single-colour images. (d) Upregulation of CD24 during mitosis as revealed by western blot of cellular lysates prepared from nocodazale-synchronized DU145 cells. (e) Diagram of CD24-GFP and GFP-CD24 constructs. The N-terminus-tagged CD24 was produced by inserting the GFP-coding sequence after the signal peptide, whereas the C-terminus-tagged CD24 was generated by inserting the GFP-coding sequence before the stop codon of CD24. (f) Tagging the C-terminus with GFP prevents cell surface localization of CD24. The images show the distinct distribution of green fluorescence in cells transfected with either CD24-GFP (C) or GFP-CD24 (N). (g) Verification of cell surface versus intracellular CD24 expression by cell surface staining. CD24-GFP (C) was not present on the surface of DU145 cells as it was not detected by an anti-CD24 mAb added to non-permeabilized cells. CD24-GFP (N) was used as positive control for cell surface CD24. (h) Verification of fusion protein expression by western blot using anti-CD24 and anti-GFP antibodies. (i) Intracellular CD24 encoded by CD24-GFP (C) is at least as potent in promoting proliferation of DU145 cells ad GFP-CD24 (N). CD24-silenced DU145 cells were transfected with CD24-GFP (C) or GFP-CD24 (N) plasmids. After drug selection, an equal number of drug-resistant transfectants were plated onto 10-cm plates. The colonies were stained with crystal violet. All images have been reproduced three times. Figure 5: Intracellular CD24 and proliferation of prostate cancer cells. ( a ) Measurement of cell surface and total cellular CD24 by flow cytometry. The prostate cancer cell lines PC3, DU145 and LNCaP were stained with anti-CD24 with or without permeabilization to measure either cell surface (top) or total cellular CD24 (bottom). ( b ) Analysis of CD24 in the cytoplasmic and plasma membrane fraction (Cp+Cm), nucleoplasm (Np) and the insoluble fraction that includes chromatin by western blot. The efficiency of the fractionation was monitored by the presence of β-actin (Cp+Cm+Np), Lamin (Np) and H1.5 (chromatin). ( c ) Confocal microscopy reveals dynamic upregulation and localization of CD24 during mitosis. Note alterations of CD24 distribution and signal intensity at different phases during mitosis. See Supplementary Fig. 6 for single-colour images. ( d ) Upregulation of CD24 during mitosis as revealed by western blot of cellular lysates prepared from nocodazale-synchronized DU145 cells. ( e ) Diagram of CD24-GFP and GFP-CD24 constructs. The N-terminus-tagged CD24 was produced by inserting the GFP-coding sequence after the signal peptide, whereas the C-terminus-tagged CD24 was generated by inserting the GFP-coding sequence before the stop codon of CD24. ( f ) Tagging the C-terminus with GFP prevents cell surface localization of CD24. The images show the distinct distribution of green fluorescence in cells transfected with either CD24-GFP (C) or GFP-CD24 (N). ( g ) Verification of cell surface versus intracellular CD24 expression by cell surface staining. CD24-GFP (C) was not present on the surface of DU145 cells as it was not detected by an anti-CD24 mAb added to non-permeabilized cells. CD24-GFP (N) was used as positive control for cell surface CD24. ( h ) Verification of fusion protein expression by western blot using anti-CD24 and anti-GFP antibodies. ( i ) Intracellular CD24 encoded by CD24-GFP (C) is at least as potent in promoting proliferation of DU145 cells ad GFP-CD24 (N). CD24-silenced DU145 cells were transfected with CD24-GFP (C) or GFP-CD24 (N) plasmids. After drug selection, an equal number of drug-resistant transfectants were plated onto 10-cm plates. The colonies were stained with crystal violet. All images have been reproduced three times. Full size image Next, we tagged CD24 at the C- and N-termini to study its localization ( Fig. 5e ). Interestingly, tagging CD24 at the C-terminus prevented its localization to the cell surface, whereas tagging the N-terminus of mature CD24 protein resulted in plasma membrane and intracellular localization, as shown in Fig. 5f . The intracellular distribution of CD24-GFP (C) was confirmed by staining non-permeabilized cells with an anti-CD24 monoclonal antibody ( Fig. 5g ). Moreover, CD24 was expressed as GFP fusion proteins, as they reacted with both anti-GFP and anti-CD24 antibodies by western blot analysis ( Fig. 5h ). Notably, CD24-GFP (N) was considerably more heterogeneous than CD24-GFP (C), reflecting its heterogeneous glycosylation status compared with CD24-GFP (C). To determine whether the intracellular form was sufficient to promote tumour cell growth, we used genetic complementation to confirm that the impact of gene silencing was attributable to CD24. We reconstituted CD24-silenced DU145 cells with either CD24-GFP (C) or GFP-CD24 (N) and monitored the impact of CD24 on tumour cell proliferation in vitro . As shown in Fig. 5i , the intracellular form of CD24, CD24-GFP (C), was at least as potent as CD24-GFP (N) in promoting tumour cell growth. CD24 silencing also reduced the growth of PC3 cells ( Supplementary Fig. 7 ). As CD24 is expressed only intracellularly in PC3 cells, its contribution to PC3 growth suggests that intracellular CD24 is sufficient to promote cancer cell proliferation. Taken together, the data presented in this section demonstrate that intracellular CD24 is sufficient to promote tumour cell proliferation. CD24 competes with ARF for binding to NPM In order to understand how CD24 encourages cancer cell growth, we identified CD24-associated proteins by mass spectrometric analysis of trypsin-digested anti-CD24 immunoprecipitates from WT but not CD24-deficient spleen cells [48] . We identified 12 unique NPM peptides in immunoprecipitates from Cd24 +/+ spleen cells and none from Cd24 −/− spleen cells ( Supplementary Table 2 ). These data suggest that CD24 may interact with NPM. NPM is a nucleolar protein and forms a punctate structure in the nucleus that dispersed during mitosis. Interestingly, the CD24–NPM association occurred transiently during mitosis. CD24 was more broadly distributed than NPM at the interphase ( Fig. 6a ), although some overlap between the two signals can also be observed ( Fig. 6b ). However, at metaphase and anaphase, CD24 and NPM were largely co-localized ( Fig. 6a,b ; see also Supplementary Fig. 8 for single-colour images). To confirm this observation in human tumour cells, we immunoprecipitated CD24 from DU145 cells and probed them with an anti-NPM monoclonal antibody. As shown in Fig. 6c , anti-CD24 co-precipitated NPM. Conversely, anti-NPM co-precipitated CD24. To map the region in NPM that interacts with CD24, we used a series of Myc-tagged deletion mutants of NPM and HA-tagged CD24. As shown in Fig. 6d , full-length (1–294) and all but one (AA1-177) truncation mutant co-precipitated CD24. As a small NPM C-terminal only fragment encompassing AA196-294 co-precipitated CD24, CD24 interacts with the C-terminus of NPM. However, as the AA196-294 fragment showed reduced association compared with the AA117-294 fragment, a contribution of the NPM core region to the interaction cannot be ruled out. 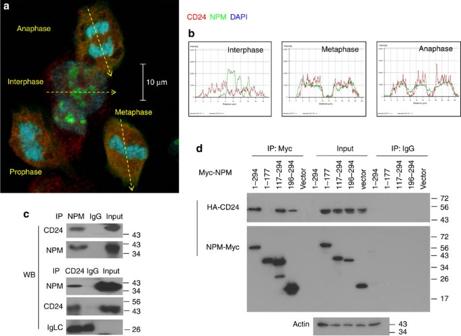Figure 6: CD24 interacts with NPM during mitosis. (a,b) Dynamic association between CD24 and NPM in DU145 cells. (a) Merged images displaying DNA (stained with DAPI, blue), NPM (green) and CD24 (red). Cells at prophase, metaphase and anaphase were identified by their chromatin distribution. The representative image was obtained from a Meta laser-scanning confocal microscope. (b) Overlay between CD24 (red) and NPM (green) signals of cells at the three indicated phases during mitosis. The intensity (yaxis) of signals was simultaneously obtained from the laser-scanning cross-section with the major diameter and overlap of the red and the green signals was analysed using LSM image browser. (c) Reciprocal co-precipitation between CD24 and NPM in DU145 cells. The cells lysates were prepared after 2 h of release from nocodazale arrest. The cell lysates were precipitated with antibodies specific for either NPM or CD24 or IgG control. The precipitates were probed by western blot with indicated antibodies. (d) Localizing the CD24-binding domain in NPM to the regions of AA196-294 based on co-IP of Myc-tagged NPM fragments and HA-tagged CD24 in HA-CD24 and NPM-Myc co-transfected HEK293 cells. The association was confirmed by western blot with anti-HA and anti-Myc mAbs. All images have been reproduced three times. DAPI, 4',6-diamidino-2-phenylindole. Co-IP, co-immunoprecipitation; IgLC, immunoglobulin light chain; IP, immunoprecipitation; IB, immunoblot. Figure 6: CD24 interacts with NPM during mitosis. ( a , b ) Dynamic association between CD24 and NPM in DU145 cells. ( a ) Merged images displaying DNA (stained with DAPI, blue), NPM (green) and CD24 (red). Cells at prophase, metaphase and anaphase were identified by their chromatin distribution. The representative image was obtained from a Meta laser-scanning confocal microscope. ( b ) Overlay between CD24 (red) and NPM (green) signals of cells at the three indicated phases during mitosis. The intensity ( y axis) of signals was simultaneously obtained from the laser-scanning cross-section with the major diameter and overlap of the red and the green signals was analysed using LSM image browser. ( c ) Reciprocal co-precipitation between CD24 and NPM in DU145 cells. The cells lysates were prepared after 2 h of release from nocodazale arrest. The cell lysates were precipitated with antibodies specific for either NPM or CD24 or IgG control. The precipitates were probed by western blot with indicated antibodies. ( d ) Localizing the CD24-binding domain in NPM to the regions of AA196-294 based on co-IP of Myc-tagged NPM fragments and HA-tagged CD24 in HA-CD24 and NPM-Myc co-transfected HEK293 cells. The association was confirmed by western blot with anti-HA and anti-Myc mAbs. All images have been reproduced three times. DAPI, 4',6-diamidino-2-phenylindole. Co-IP, co-immunoprecipitation; IgLC, immunoglobulin light chain; IP, immunoprecipitation; IB, immunoblot. Full size image CD24 alleviates tumour-suppressor activity of p14ARF To determine whether CD24 competes with ARF for interaction with NPM, we co-incubated recombinant ARF with either control glutathione S -transferase (GST) or NPM–GST in the presence of increasing amounts of CD24-Fc or control IgG-Fc. The proteins that associated with the GST-fusion proteins were pulled down using glutathione beads and identified by western blot using anti-NPM, anti-CD24 or anti-ARF. As shown in Fig. 7a , CD24-Fc, but not control IgG-Fc, blocked the ARF–NPM association in a dose-dependent manner. To determine whether CD24 inhibits the ARF–NPM association in cancer cells, we used a proximity ligation assay to assess the association between NPM and ARF in DU145 cells with or without CD24 silencing. A summary of three experiments is shown in Fig. 7b , whereas representative images from one experiment are shown in Fig. 7c . These data demonstrate that shRNA silencing of CD24 increased the NPM–ARF association in tumour cells. To test if CD24 also affects the ARF–NPM interaction in normal cells, we compared the amounts of Npm-associated Arf in WT and Cd24 −/− thymocytes. As shown in Fig. 7d , a substantial increase in Npm-associated Arf was observed in Cd24 −/− thymocytes. These results demonstrate that CD24 inhibited ARF association with NPM. 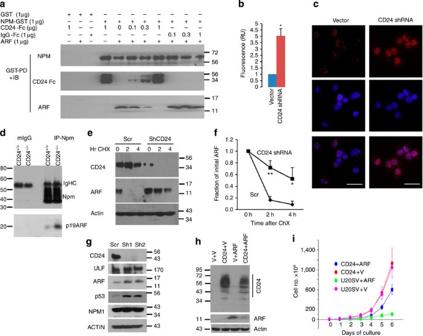Figure 7: CD24 inhibits tumour-suppressor activity of ARF by antagonizing the NPM–ARF interaction. (a) Recombinant CD24 associates with recombinant NPM and blocks the ARF–NPM interaction. Control GST and NPM–GST fusion proteins were incubated with indicated amounts of CD24-Fc and/or ARF. The GST or GST–NPM1-associated proteins were determined by western blot after pull-down with glutathione beads. (b,c) Proximity ligation assay reveals CD24 antagonism of NPM–ARF association. Scrambled orCD24 shRNA-transduced DU145 cells were compared for endogenous NPM–ARF association. Images were obtained using an Olympus BX61 microscope using a × 60 oil objective. Scale bar, 50 μm. Image J software was used to quantify fluorescent intensities. Mean fluorescent intensities were determined from more than 100 cells per slide. This experiment has been repeated three times. Data shown are means and s.d. of three independent repeats (b) and representative images (c). (d) Cd24 reduces Npm-associated p19Arf. Spleen lysates from WT andCd24−/−mice were precipitated with anti-Npm mAb. The amounts of Npm and p19Arf in the immunoprecipitates were determined by western blot. IgG heavy chain (IgHC) was used as loading controls. (e) Regulation of ARF levels and stability by endogenous CD24. Scrambled or shRNA-silenced DU145 cells were arrested at G2/M phase overnight and then treated with CHX for 0, 2 and 4 h. The levels of CD24 (upper panel) and p14ARF were analysed by western blot. (f) Decay kinetics of p14ARF are shown as % of ARF protein at different times after CHX treatment. (g) ShRNA silencing ofCD24does not affect the levels of the ARF E3 ligase ULF. (h) Ectopic expression of CD24 reduces ARF levels. U2OS cells that ectopically expressedCD24alone,ARFalone or both were analysed for their CD24 and ARF levels by western blot. (i) CD24 expression alleviates ARF tumour-suppressor activity. Data shown are growth kinetics of U2OS cells transfected with the given plasmids. Data shown are means and s.d. of cell numbers during the 6-day period. All data in this figure have been reproduced two or three times. Figure 7: CD24 inhibits tumour-suppressor activity of ARF by antagonizing the NPM–ARF interaction. ( a ) Recombinant CD24 associates with recombinant NPM and blocks the ARF–NPM interaction. Control GST and NPM–GST fusion proteins were incubated with indicated amounts of CD24-Fc and/or ARF. The GST or GST–NPM1-associated proteins were determined by western blot after pull-down with glutathione beads. ( b , c ) Proximity ligation assay reveals CD24 antagonism of NPM–ARF association. Scrambled or CD24 shRNA -transduced DU145 cells were compared for endogenous NPM–ARF association. Images were obtained using an Olympus BX61 microscope using a × 60 oil objective. Scale bar, 50 μm. Image J software was used to quantify fluorescent intensities. Mean fluorescent intensities were determined from more than 100 cells per slide. This experiment has been repeated three times. Data shown are means and s.d. of three independent repeats ( b ) and representative images ( c ). ( d ) Cd24 reduces Npm-associated p19Arf. Spleen lysates from WT and Cd24 −/− mice were precipitated with anti-Npm mAb. The amounts of Npm and p19Arf in the immunoprecipitates were determined by western blot. IgG heavy chain (IgHC) was used as loading controls. ( e ) Regulation of ARF levels and stability by endogenous CD24. Scrambled or shRNA-silenced DU145 cells were arrested at G2/M phase overnight and then treated with CHX for 0, 2 and 4 h. The levels of CD24 (upper panel) and p14ARF were analysed by western blot. ( f ) Decay kinetics of p14ARF are shown as % of ARF protein at different times after CHX treatment. ( g ) ShRNA silencing of CD24 does not affect the levels of the ARF E3 ligase ULF. ( h ) Ectopic expression of CD24 reduces ARF levels. U2OS cells that ectopically expressed CD24 alone, ARF alone or both were analysed for their CD24 and ARF levels by western blot. ( i ) CD24 expression alleviates ARF tumour-suppressor activity. Data shown are growth kinetics of U2OS cells transfected with the given plasmids. Data shown are means and s.d. of cell numbers during the 6-day period. All data in this figure have been reproduced two or three times. Full size image As NPM enhances ARF stability, we next tested if shRNA silencing of the CD24 gene increases ARF stability and accumulation using G2-M-arrested DU145 cells. In order to observe CD24-dependent changes on steady-state levels of ARF without the influx of new protein synthesis, we treated G2-M-arrested cells with cycloheximide (CHX) and measured ARF levels at 0, 2 and 4 h after CHX treatment. As shown in Fig. 7e,f , in comparison to Scr shRNA-transfected cells, CD24 shRNA-transfected cells markedly increased ARF protein levels at time 0. Moreover, although ARF was clearly detectable at 4 h after CHX treatment in CD24-silenced DU145 cells, very little (if any) ARF was detected in Scr shRNA-transduced control cells 2 h after CHX treatment. Chen et al . [49] reported that the ARF–NPM interaction in the nucleolus prevented ULF-mediated ARF degradation in the nucleoplasm. We compared ULF levels in DU145 cells with or without CD24 silencing and found that ULF was unaffected by CD24 silencing ( Fig. 7g ). Therefore, CD24 regulated ARF levels by reducing NPM–ARF association rather than through increasing the levels of the ubiquitin ligase ULF. To determine whether CD24 promotes tumour cell growth by antagonizing ARF function, we introduced ARF and/or CD24 into the ARF-deficient U2OS cell line [50] . As shown in Fig. 7h , ectopic expression of CD24 reduced ARF levels. More importantly, CD24 bypassed ARF-mediated growth inhibition but had no effect in ARF-null cells ( Fig. 7i ). Therefore, CD24 promotes tumour growth by antagonizing ARF function. ShRNA silencing of CD24 restores mutant p53 function Given the effect of ARF on MDM2 and its substrate p53, we evaluated if CD24 affected the expression of MDM2 and p53 in an ARF-dependent manner. As shown in Fig. 8a , in ARF-expressing DU145 cells, CD24 silencing increased the levels of ARF and p53 and reduced that of MDM2. Elevated ARF levels contributed to CD24-mediated reduction of MDM2 and p53 as CD24 had no effect on the levels of MDM2 and p53 in ARF-deficient U2OS cells ( Fig. 8b ). Furthermore, expression of p21 following shRNA silencing of CD24 was due to elevated p53 levels as shRNA silencing of p53 in DU145 cells substantially reduced p21 levels ( Fig. 8c ). 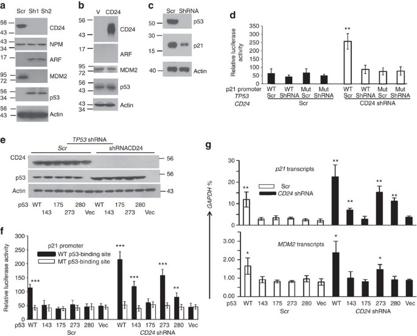Figure 8: CD24 silencing restores transcriptional activity of p53. (a) Effect of CD24 silencing on expression of NPM, ARF, MDM2 and p53. Scrambled (Scr) orCD24-shRNA-silenced DU145 cells were analysed for CD24, NPM, ARF, MDM2 and p53 by western blot. (b) In ARF-deficient U2OS cells, ectopic expression of CD24 had no effect on the levels of MDM2 and p53. Actin levels were used as loading control. (c) Endogenous mutant p53 is responsible for the upregulation of p21 in CD24-silenced DU145 cells. (d) In DU145 cells, silencingCD24restores transcriptional induction of the p21 promoter. DU145 cells transduced with Scr or shRNA for eitherTP53orCD24were transfected with a luciferase reporter containing the p21 promoter. The WT reporter has an intact p53-binding site, whereas the mutant promoter has the site deleted. (e,f) CD24 silencing restores transcriptional activity of multiple TP53 mutants. DU145 cells in which the endogenousTP53was silenced by shRNA were transduced with Scr or CD24 shRNA lentivirus. The stable cell lines were then transfected with p53 mutants in conjunction with WT or mutant p21 promoter reporter constructs. p53 levels (e) were determined by western blot, while luciferase activity (f) was measured at 72 h after transfection. The mutants used were p53R273H, p53V143A, p53R280Tand p53R175H. Numbers on thexaxis indicate the amino-acid positions of the p53 mutations. (g) As ineandf, except that the endogenous p21 and MDM2 mRNA were measured by quantitative PCR. Data shown are means and s.d. of triplicate samples. All data have been reproduced two or three times. Figure 8: CD24 silencing restores transcriptional activity of p53. ( a ) Effect of CD24 silencing on expression of NPM, ARF, MDM2 and p53. Scrambled (Scr) or CD24 -shRNA-silenced DU145 cells were analysed for CD24, NPM, ARF, MDM2 and p53 by western blot. ( b ) In ARF-deficient U2OS cells, ectopic expression of CD24 had no effect on the levels of MDM2 and p53. Actin levels were used as loading control. ( c ) Endogenous mutant p53 is responsible for the upregulation of p21 in CD24-silenced DU145 cells. ( d ) In DU145 cells, silencing CD24 restores transcriptional induction of the p21 promoter. DU145 cells transduced with Scr or shRNA for either TP53 or CD24 were transfected with a luciferase reporter containing the p21 promoter. The WT reporter has an intact p53-binding site, whereas the mutant promoter has the site deleted. ( e , f ) CD24 silencing restores transcriptional activity of multiple TP53 mutants. DU145 cells in which the endogenous TP53 was silenced by shRNA were transduced with Scr or CD24 shRNA lentivirus. The stable cell lines were then transfected with p53 mutants in conjunction with WT or mutant p21 promoter reporter constructs. p53 levels ( e ) were determined by western blot, while luciferase activity ( f ) was measured at 72 h after transfection. The mutants used were p53 R273H , p53 V143A , p53 R280T and p53 R175H . Numbers on the x axis indicate the amino-acid positions of the p53 mutations. ( g ) As in e and f , except that the endogenous p21 and MDM2 mRNA were measured by quantitative PCR. Data shown are means and s.d. of triplicate samples. All data have been reproduced two or three times. Full size image DU145 cells harbour a bi-allelic missense mutation of TP53 (ref. 51 ; (p53 223L and p53 274F ). Both mutants exhibit tumour-suppressor activity based on the cellular context and culture conditions [52] , [53] . As the molecular basis of this context-dependent tumour-suppressor activity is unknown, we tested whether CD24 determines the function of the mutant p53. We used two luciferase reporter constructs driven by the p21 promoter with a p53 consensus binding site (wt/WWP-luc) or without a p53-binding site (mu/DW-luc) [54] . The p53-dependent activity was further evaluated by transfection of an shRNA-targeting endogenous p53. As shown in Fig. 8d , in CD24-expressing DU145 cells, no endogenous p53 activity was detected, as basal levels of p21 promoter activity were observed regardless of a p53-binding site or p53 silencing. In contrast, shRNA silencing of CD24 resulted in a dramatic increase in p21 promoter activity. The activity was entirely dependent on (i) the p53-binding site and (ii) the endogenous p53 protein itself, as an induction was not observed in the luciferase reporter driven by the p21 promoter with the p53 site deleted (mut) or was abrogated upon transfection of a p53-targeting shRNA ( Fig. 8d ). Thus, upregulation of p53 induced by CD24 silencing was causally related to increased p21 expression in DU145 cells. To determine the functional impact of CD24 on commonly occurring cancer-associated p53 mutants, we ectopically expressed TP53 mutants in the DU145 cell line that had been depleted of endogenous p53, using a p53 shRNA specific for endogenous TP53 via 3′ untranslated region (UTR) targeting, thus sparing the mutant TP53 cDNA (complementary DNA) lacking the 3′UTR. As expected, CD24 silencing increased accumulation of mutant p53 protein ( Fig. 8e ). The function of the TP53 mutants was measured based on transactivation of the p21 promoter with or without a p53-binding site. As expected, in the absence of exogenous TP53 cDNA, the luciferase activity of both promoters was unaffected by mutation of the p53-binding sites, regardless of whether the endogenous CD24 gene was silenced ( Fig. 8f ). These data show effective silencing of the endogenous TP53. Surprisingly, shRNA silencing of CD24 increased activities of WT as well as three of the four TP53 mutants, including the p53 R273H mutant, the most common TP53 mutation, and p53 V143A and p53 R280T . The other common mutant, p53 R175H , which causes a conformational change in p53, remained inactive regardless of CD24 status ( Fig. 8f ). Consistent with the reporter assays, silencing CD24 allowed significant induction of p21 mRNA by p53 R273H , p53 V143A and p53 R280T , but not p53 R175H ( Fig. 8g ). Interestingly, the impact of CD24 was not uniform to all p53 target genes. As shown in Fig. 8f , with the exception of a moderate effect of p53 R273H , none of the TP53 mutants tested significantly induced expression of the endogenous MDM2 gene. The lack of MDM2 induction explains the increased accumulation of functional p53 mutant protein after CD24 silencing ( Fig. 8a ). Although the mechanism for selective induction of p21 by the p53 mutant remains to be elucidated, selective induction of p21 has been reported in tumour cells after high doses of irradiation or undergoing chemotherapy [55] , [56] . Cd24 silencing bypasses p53 inactivation by viral oncogenes p53 protein is inactivated by SV40 T antigen and this inactivation requires interaction between p53 and SV40 T antigen [57] . To determine whether Cd24 abrogates p53 function in SV40 T antigen-induced cancer cells, we compared the SV40 TAg-transduced mouse prostate cancer cell line C3 with or without endogenous Cd24 expression. As shown in Fig. 9a , shRNA silencing of Cd24 resulted in increased p53 levels, as expected. To determine whether the increased p53 was subjected to inactivation by SV40 T antigen, we assessed the relative amount of SV40 T antigen-associated versus non-associated p53 in Cd24-expressing and non-expressing C3 cells. As shown in Fig. 9a , right panels, Cd24 shRNA silencing resulted in a massive increase of SV40 T antigen-free p53, although a small increase in SV40 T antigen-associated p53 was also observed. As CD24 was not co-precipitated with SV40 T antigen, it is likely that the primary function of CD24 is to decrease p53 levels. Consistent with inactivation of p53 by large T antigen in CD24-expressing C3 cells, the p21 promoter was largely inactive in the scrambled shRNA-transduced C3 cells ( Fig. 9b , top panel). Importantly, shRNA silencing of Cd24 caused a major increase in p21 promoter activity ( Fig. 9b , top panel). This increase was fully attributable to p53 as it required a p53-binding site on the p21 promoter and was abrogated by shRNA silencing of TP53 ( Fig. 9b , top panel). We compared the levels of p21 and p53 in prostate cancer from Cd24 +/+ , Cd24 +/− and Cd24 −/− TRAMP mice by immunohistochemistry (IHC). The tumour cells in this model have WT TP53 (ref. 58 ). As shown in Fig. 9c , Cd24 +/− and Cd24 −/− prostate cancers showed considerably higher levels of p53 and p21 than the WT prostate cancer. 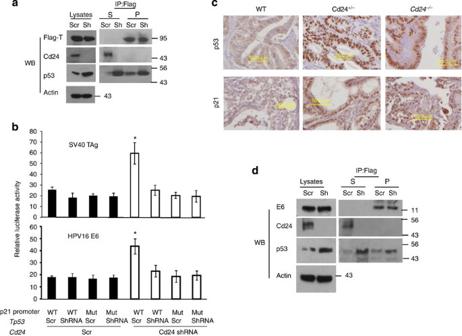Figure 9: CD24 is required for viral oncogene-mediated inactivation of p53 function. (a) By increasing the overall levels of p53 protein,Cd24silencing increases the proportion of SV40 T antigen-unbound p53. SV40 T antigen was tagged with Flag and introduced into the mouse prostate cancer cell line C3 with or without transduction of CD24 shRNA. The total cellular (left panel) or SV40 T antigen-associated or non-associated p53 (right panel) were determined by either western blot or anti-Flag immunoprecipitation followed by western blot. Note that CD24 was not co-precipitated. S: supernatant; P: pellet. (b) Cd24 silencing reveals p53 function in SV40 large T antigen (SV40 Tag)-transduced (top) and human papilloma viral protein E6 (HPV E6)-transduced C3 cells (bottom). SV40 Tag- or HPV E6-transduced C3 cells were transfected with WT or p53-binding site mutant p21 promoter linked with a luciferase reporter. The function of the endogenousCd24andTp53locus was confirmed by shRNA silencing of either genes. Data shown are means and s.d. of relative luciferase activity. (c) In theTp53+/+TRAMP model, targeted mutation ofCd24increased the levels of p53 and p21. Data shown are photographs of immunohistochemical analysis of p21 and p53 levels from eitherCd24+/+orCd24−/−prostate cancer samples. (d)Cd24silencing increases the proportion of HPV E6-unbound p53, as ina, except that HPV E6 was used instead of SV40 TAg. All data in this figure have been reproduced two or three times. Co-IP, co-immunoprecipitation; Mut, mutant; WB, western blot. Figure 9: CD24 is required for viral oncogene-mediated inactivation of p53 function. ( a ) By increasing the overall levels of p53 protein, Cd24 silencing increases the proportion of SV40 T antigen-unbound p53. SV40 T antigen was tagged with Flag and introduced into the mouse prostate cancer cell line C3 with or without transduction of CD24 shRNA. The total cellular (left panel) or SV40 T antigen-associated or non-associated p53 (right panel) were determined by either western blot or anti-Flag immunoprecipitation followed by western blot. Note that CD24 was not co-precipitated. S: supernatant; P: pellet. ( b ) Cd24 silencing reveals p53 function in SV40 large T antigen (SV40 Tag)-transduced (top) and human papilloma viral protein E6 (HPV E6)-transduced C3 cells (bottom). SV40 Tag- or HPV E6-transduced C3 cells were transfected with WT or p53-binding site mutant p21 promoter linked with a luciferase reporter. The function of the endogenous Cd24 and Tp53 locus was confirmed by shRNA silencing of either genes. Data shown are means and s.d. of relative luciferase activity. ( c ) In the Tp53 +/+ TRAMP model, targeted mutation of Cd24 increased the levels of p53 and p21. Data shown are photographs of immunohistochemical analysis of p21 and p53 levels from either Cd24 +/+ or Cd24 −/− prostate cancer samples. ( d ) Cd24 silencing increases the proportion of HPV E6-unbound p53, as in a , except that HPV E6 was used instead of SV40 TAg. All data in this figure have been reproduced two or three times. Co-IP, co-immunoprecipitation; Mut, mutant; WB, western blot. Full size image Human papilloma viruses (HPVs) 16 and 18 are now well-established causes for human cancer [59] , [60] . It has been demonstrated that the viral E6 oncogenes associates with p53 to inactivate its tumour-suppressor activity [61] . To determine whether CD24 is required for E6-mediated p53 inactivation, we transduced HPV16 E6 gene into the C3 cell line (C3-E6), and compared the levels of p53 in Scr or Cd24 shRNA-silenced C3-E6 cells. As shown in Fig. 9d , Cd24 -silencing increased p53 levels in the C3-E6 cells. Importantly, most of the increased p53 was not associated with E6 ( Fig. 9d ). Corresponding to increased E6-unbound p53, a significant increase in p21 promoter activity was observed after CD24 silencing ( Fig. 9b , lower panel). CD24 silencing reactivates mutant p53 We tested the effect of WT and mutant p53 for their inhibition of proliferation of Scr or CD24 shRNA-transduced DU145 cells. Endogenous p53 was removed by an shRNA targeting the 3′ UTR of the TP53 gene. The cDNAs for WT and mutant p53 (lacking 3′ UTR) were introduced into either Scr or CD24 shRNA viral vector-transduced cell lines. WT p53 suppressed growth of DU145 regardless of CD24 expression. In the Scr shRNA transfectants, none of the mutants greatly reduced the colony number or size, as expected. A general but moderate reduction in colony numbers by all mutants was observed, which is likely due to more efficient expression of the drug-resistance gene in the vector devoid of p53 insert. In CD24-silenced DU145 cells, however, p53 R273H was almost as efficient as WT p53 in suppressing colony formation. The p53 V143A and p53 R280T mutants were also significantly more efficient in suppressing proliferation of cells that were silenced of the CD24 gene, although CD24 silencing did not confer tumour-suppressor activity to p53 R175H . The above data suggested that for a high proportion of p53 mutations, CD24 expression may be a necessary co-factor in cancer development. To explore this possibility, we searched the Cancer Genome Atlas (TCGA) database for a possible association between CD24 overexpression and TP53 mutation in cancer samples. We limited our search to cohorts that meet two criteria. First, both RNAseq and p53 status data are available. Second, the Cd24 RNA levels must show a broad distribution. Three cohorts, including low-grade glioma, glioblastoma and prostate cancer, satisfied both criteria. We divided the cancer samples into CD24 hi (with CD24 mRNA above the median) and CD24 lo (with CD24 mRNA below the median) and compared the mutation rates. As shown in Fig. 10c , in all three cancer types, we observed a significantly higher rate of TP53 mutation among the CD24 hi groups. Based on odds ratio, the mutations TP53 were two to four times more likely to occur in CD24 hi group. The association was not due to leukocyte infiltration as the RNA for CD45, a pan-leukocyte marker, did not correlate with either CD24 levels or TP53 mutation rate ( Supplementary Fig. 9 ). 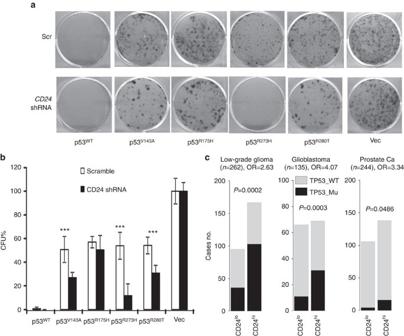Figure 10: ShRNA silencing of CD24 restores tumour-suppressor activity of cancer-associated p53 mutants. (a) DU145 cells whose endogenous TP53 was silenced were transduced with cDNAs of cancer-associated p53 mutants used inFig. 8e,fand then cultured in six-well plates in the presence of neomycin for 2 weeks before the colonies were photographed and counted. Representative image of each transfectant is shown. (b) ShRNA silencing of CD24 reactivates the tumour-suppressor activity of p53R273Has assessed by the number of DU145 colonies visualized by crystal violet. Data shown are means and s.d. of triplicate samples and have been normalized against the vector control (artificially defined as 100%) from DU145 cells transduced with either Scr or CD24 ShRNA. The data have been reproduced twice. (c)In silicoanalysis revealed an association between CD24 levels and TP53 status. The expression and mutational status data were obtained from the TCGA database as detailed in the Methods section. Glioblastoma, low-grade brain glioma and prostate cancer samples were divided into CD24hi(above the mean) and CD24lo(below the mean) groups based on RNA-seq data. The frequencies of the samples with somatic Tp53 mutations were compared using either Pearson’sχ2tests with correction for low counts of mutant samples in the prostate cancer cohort. CFU, colony-forming unit. Figure 10: ShRNA silencing of CD24 restores tumour-suppressor activity of cancer-associated p53 mutants. ( a ) DU145 cells whose endogenous TP53 was silenced were transduced with cDNAs of cancer-associated p53 mutants used in Fig. 8e,f and then cultured in six-well plates in the presence of neomycin for 2 weeks before the colonies were photographed and counted. Representative image of each transfectant is shown. ( b ) ShRNA silencing of CD24 reactivates the tumour-suppressor activity of p53 R273H as assessed by the number of DU145 colonies visualized by crystal violet. Data shown are means and s.d. of triplicate samples and have been normalized against the vector control (artificially defined as 100%) from DU145 cells transduced with either Scr or CD24 ShRNA. The data have been reproduced twice. ( c ) In silico analysis revealed an association between CD24 levels and TP53 status. The expression and mutational status data were obtained from the TCGA database as detailed in the Methods section. Glioblastoma, low-grade brain glioma and prostate cancer samples were divided into CD24 hi (above the mean) and CD24 lo (below the mean) groups based on RNA-seq data. The frequencies of the samples with somatic Tp53 mutations were compared using either Pearson’s χ 2 tests with correction for low counts of mutant samples in the prostate cancer cohort. CFU, colony-forming unit. Full size image A recent meta-analysis of immunohistochemistry data between 1990 and 2009 revealed that CD24 is expressed in 68% of clinical samples across all major cancer types [62] . A major challenge in understanding the oncogenic function of CD24 is to establish a central programme determining how CD24 promotes oncogenesis. Our data reveal a critical role for intracellular CD24 in tumour cell growth. A mass spectrometry-based approach led to the identification of a CD24–NPM interaction. This interaction occurred endogenously was direct as it was recapitulated with recombinant CD24-Fc and NPM–GST fusion proteins. Interestingly, the association between CD24 and NPM was most prominent during metaphase and anaphase of mitosis. As such, it is intriguing to consider whether CD24 function may be more prominent during mitosis. In vitro analysis with recombinant CD24, ARF and NPM provided definitive evidence that CD24 prevents ARF from interacting with NPM. Being largely unstructured, ARF is known to be rapidly degraded unless associated with NPM [63] . The idea that CD24 promotes tumour growth by causing ARF degradation is supported by the fact that ectopic expression of CD24 bypassed ARF-mediated suppression of growth of cancer cells. CD24 had no impact on the growth rate in ARF-deficient U2OS cells, further supporting the concept that CD24 transforming potential is mediated through ARF. Therefore, a central function of CD24 in cancer cells may be to inhibit the ARF–NPM interaction, thereby causing ARF degradation. This degradation results in increased MDM2 levels that subsequently reduced p53 levels. Although immunofluorescence staining suggests that the CD24–NPM association was most prominent at M phase, dispersion of NPM and increased expression of CD24 may have facilitated observation of CD24–NPM co-localization during mitosis. A modest but clear co-localization can be found in non-mitotic cells. Consistent with this notion, we observed localization of CD24 in the nucleoli ( Supplementary Fig. 10 ). Therefore, in fact, the association between CD24 and NPM can be easily detected by co-immunoprecipitation in cells that have exited from mitosis. Consistent with this view, the impact of CD24 silencing on NPM-associated ARF was clearly demonstrable among mostly non-mitotic thymocytes. In addition, proximity ligation assay revealed that CD24 silencing increased the NPM–ARF association in non-mitotic DU145 cells. Furthermore, silencing CD24 increased ARF, p21 and p53 while reducing MDM2 in non-synchronized DU145 cells. Oncogenic insults often leads to activation of ataxia telangiectasia mutated (ATM) [64] . As ATM activation has been shown to be associated with reduced ARF–NPM association [65] , it is of interest to determine whether CD24 activates ATM. As shown in Supplementary Fig. 11 , using p-Ser1981-specific antibodies as indicator for ATM activation, we found no evidence of increased ATM activation in the CD24-expressing DU145 cells. Previous studies indicate that many of the TP53 mutants, including nearly 50% of the p53 mutations in glioblastoma, are temperature sensitive [44] . Here, we showed that in DU145 cells, which harbour such a temperature-sensitive mutation, shRNA silencing of CD24 prevented mutational inactivation of TP53 . In addition, CD24 silencing at least partially restored transcriptional activity of three out of four cancer-associated p53 mutants, including the most common R273H mutation. These data support the idea that although not all cancer samples require CD24 for genetic inactivation of p53, CD24 is a major necessary cellular component associated with many inactivating p53 mutations in cancer. Furthering this concept, we observed that in cancers with heterogeneity in CD24 transcripts, the TP53 mutation rate was significantly higher among those samples with higher levels of CD24 transcripts. In addition, our data revealed that by regulating p53 levels, CD24 also determines the susceptibility of p53 to inactivation by viral oncogenes, such as the SV40 large T Ag and HPV16 E6-antigen. Therefore, by decreasing p53 protein levels, CD24 allows inactivation of p53 activity by both mutation and viral oncogenes. It should be noted that since ARF is known to suppress tumour development even in the Tp53 −/− mice, it is anticipated that CD24, being a regulator of ARF degradation, should also function in a p53-independent manner. Although the mechanism of p53-independent pro-tumorigenic actions of CD24 remains to be determined, our data support this idea by showing that CD24 silencing also suppresses the growth of p53-null PC3 cells. Based on the data presented, we propose a mechanism by which intracellular CD24 regulates cancer pathogenesis. By inhibiting ARF binding to NPM, intracellular CD24 causes ARF destabilization that subsequently increases in MDM2 and decreases p53 and p21. Our model provides a convergent explanation for three mysteries in cancer pathogenesis: the broad upregulation of CD24, the predominance of TP53 missense mutations and the apparent lack of ARF-specific mutations [2] , [37] . Additional studies in more tumour models will be needed to determine whether the concept is generally applicable. Finally, as p53 is among the most commonly inactivated tumour suppressors, a major challenge in tumour therapy is how to restore p53 tumour-suppressor activity. In this context, we showed that in addition to the endogenously expressed temperature-sensitive mutant in DU145 cells, silencing CD24 also restores at least part of the tumour-suppressor activity of three out of four p53 mutants, including the most commonly observed p53 R273H mutant. Our data provide a potential approach to restore p53 function in cancer. Experimental animals Male TRAMP mice in the C57BL/6 background were purchased from the Jackson Laboratory. The mice were bred at the animal facilities of the University of Michigan (Ann Arbor, MI, USA). Cd24-deficient C57BL/6 mice have been described previously [45] . Male BALB/c athymic nude or NSG mice were purchased from Charles River Laboratories. The progression of prostate cancer in the TRAMP model was measured by MRI as described previously [66] . The pathological evaluation was performed according to the Bar Harbor meeting guidelines [67] . All animal experiments were conducted in accordance with accepted standards of animal care and approved by the Institutional Animal Care and Use Committee of Children’s Research Institute at Children’s National Medical Center and the University of Michigan. Cell lines, antibodies and shRNAs Prostate cancer cell lines DU145, PC3 and LNCaP were obtained from the American Type Culture Collection. Antibodies specific for the following targets were used for this study: human CD24 (BD Pharmingen, ML5, Cat #:555426), mouse Cd24 (BD Pharmingen, M1/69, Cat #: 562360), CD24 (Santa Cruz Biotechnology, Cat #: sc-11406 and Cat #: sc-53660, and SN3b), NPM1 (Abcam, Cat #: ab10530), p14 (Santa Cruz Biotechnology, Cat #: sc-8340; Cell Signaling, Cat #:2407), p53 (Santa Cruz Biotechnology, DO-1, Cat #: sc-126; FL-393, Cat #sc-6243), MDM2 (Santa Cruz Biotechnology, Cat #: sc-7918), p21 (Cell Signaling, Cat #: 2946), p27 (Cell Signaling, Cat #: 2946), Cyclin B1 (Santa Cruz Biotechnology, Cat #: H-433), GFP (Cell Signaling, Cat #: 2946), Lamin B1 (Santa Cruz Biotechnology, sc-56145), H1.5 (Abcam ab18208), β-actin (Sigma-Aldrich, Cat #: A5441) and anti-IgG (Santa Cruz Biotechnology), phospho-ATM (Ser1981) (Rabbit mAb D6H9, Cat #5883, Cell Signaling) and ATM (Rabbit mAb D2E2, Cell Signaling, Cat #2873). The two CD24 shRNA constructs were CD24-V2LHS_71908 (Open Biosystems, Cat #: RHS4430-99291677, GenBank accession #: NM_013230 ) and CD24-V2LHS_71909 (Open Biosystems, Cat #: RHS4430-98854299, GenBank accession #: L33930 ). DU145 and PC3 cells were infected with lentivirus expressing either control shRNA or CD24 shRNA vectors. The sequence of shRNA and primers used for PCR are listed in Supplementary Table 3 . Fluorescence microscopy Rabbit anti-NPM (Cat#: sc-6013R, Santa Cruz Biotechnology), mouse anti-CD24 (ML5), mouse anti-α-tubulin, mouse anti-γ-tubulin (Sigma-Aldrich) and rat anti–α-tubulin (Chemicon) were used for immunofluorescence. The binding of antibodies to cells was visualized with secondary antibodies from Life Technologies: Alexa Fluor 568 Goat Anti-Mouse IgG (H+L) Antibody, highly cross-adsorbed (Red), Catalogue Number A-11031 and Alexa Fluor 488 Goat Anti-Rabbit IgG (H+L) Antibody, highly cross-adsorbed (Green), Catalogue Number A-11034. All images were obtained on an inverted microscope (Axiovert 100 M; Carl Zeiss MicroImaging, Inc.) with an LSM 510 Meta laser-scanning confocal module (Carl Zeiss MicroImaging, Inc.). Samples were scanned with appropriate lasers and filter sets and images were collected at 0.5 μm intervals using a × 63 water objective (C-Apochromat with 1.2 numerical aperture). LSM 510 Meta software (Carl Zeiss MicroImaging, Inc.) was used to collect images. Images were analysed with LSM image browser (Carl Zeiss MicroImaging, Inc.). Gene expression profiling and pathway analysis DU145 cells stably transduced with lentivirus expressing either control shRNA or CD24 shRNA were seeded onto 10-cm plates and cultured with puromycin. Individual clones were isolated and tested for CD24 expression. Clones with stable CD24 silencing were used for gene expression analysis, usually 2 months after the initial transduction. The stable clones were seeded again in 10-cm plates and at 3–5 days after culture, when the cells reached 50% confluency, the cells were washed with ice-cold PBS twice and RNA extraction was performed with the RNeasy Mini kit (Qiagen) according to the manufacturer’s protocol. Contaminated genomic DNA was eliminated with DNase I (Invitrogen) according to the manufacturer’s protocol. We conducted mRNA microarray analysis using HG-U133 Plus 2.0 (Affymeatrix) was performed according to the manufacturer’s protocol. The microarray data are submitted to NCBI GEO (accession No. GSE46708 ). dChip software (University of California at Los Angeles Clinical Microarray Core) was used to generate a heat map of the microarray profile. Gene expression profiles of cells were compared with and without CD24. Differences in mRNA expression levels between CD24 + and CD24 − cells were calculated by Student’s t -test. Ingenuity pathways analysis (IPA) for CD24-related genes was performed using IPA software (version 7.1, Ingenuity Systems, Inc.). Co-immunoprecipitation and western blot Collected cells were washed with cold PBS and lysed in ice-cold buffer (20 mM Tris–HCl (pH 8.0), 150 mM NaCl, 1 mM EDTA, 1% NP-40) supplemented with complete protease inhibitors (Sigma-Aldrich) on ice for 10 min. The samples were centrifuged at 13,000 r.p.m. for 10 min. The lysates were aliquoted into two tubes and incubated with either the designated antibody or an appropriate IgG control for 16 h at 4 °C. Protein A/G agarose (Invitrogen) was used to precipitate antibody–protein complexes. For western blotting, anti-CD24 (Santa Cruz Biotechnology, 1:1,000), anti-p27 (Cell Signaling, 1:1,000), anti-p21 (Cell Signaling, 1:1,000), anti-p53 (Santa Cruz Biotechnology, 1:2,000), anti-Lamin (Santa Cruz Biotechnology, 1:5,000), anti-H1.5 (Abcam, 1:5,000), anti-Cyclin B1 (Santa Cruz Biotechnology, 1:3,000), anti-GFP (Cell Signaling, 1:2,000), anti-NPM1 (Abcam, 1:3,000), anti-HA (Sigma-Aldrich, 1:3,000), anti-Myc (Abcam, 1:3,000), anti-ARF (Santa Cruz Biotechnology, 1:1,000), anti-MDM2 (Santa Cruz Biotechnology, 1:1,000) and anti-β-actin (Sigma, 1:5,000) antibodies were used as primary antibodies. The membranes were incubated for 1 h at room temperature in 0.25% nonfat milk with a 1:3,000–5,000 dilution of either anti-rabbit or anti-mouse IgG HRP-linked secondary antibody (Cell Signaling). Colony formation assay The colony formation assay was carried out as we have described previously [68] . DU145 or PC3 cells were transfected with either the control vector or vectors (CD24 shRNAs, CD24-EGFP-N, CD24-EGFP-C). At 48 h after transfection, cells were counted and 4 × 10 4 transfected cells were plated in 100-mm dishes in triplicate and cultured in medium containing 10 μg ml −1 puromycin. After 3 weeks in culture, the colonies were stained with 0.125% crystal violet. The colonies were either photographed or counted. The total number of colonies (≥20 cells) per plate was counted using a microscope. Xenogeneic transplantation DU145 and PC3 cells transduced with scrambled or with CD24 shRNA, or cDNA for CD24-EGFP (C), and CD24-EGFP (N) fusion proteins were grown in Eagle’s Minimum Essential Media supplemented with 10% fetal bovine serum without antibiotics. Cells were expanded and used for inoculation within three to four passages after thawing from liquid nitrogen storage. Male BALB/c athymic nude mice were obtained from Charles River Laboratories, whereas NSG mice were purchased from the Jackson Laboratories. Eight-week-old SCID mice (Jackson Laboratories) were used as recipients that received subcutaneous injections on the left flank of 100 μl containing 5 × 10 6 cells DU145 cells. Tumour size was measured using a Vernier caliper in the two longest dimensions. Tumour volume was calculated with the following formula 0.5 D 1( D 2) 2 , where D 1 is the long measure and D 2 is the short dimension. The experiments were terminated when the xenograft tumour size in the control group reached a group average calculated volume of 1 × 10 3 mm 3 . Flow cytometry For cell surface staining, cells were incubated with antibodies in staining buffer for 30 min on ice. Cells were then washed three times and fixed. For intracellular staining, cells were first fixed with Cytofix/Cytoperm buffer (BD Biosciences), followed by washing with Perm/Wash buffer (BD Biosciences), and incubated with anti-CD24 in Perm/Wash buffer for 30 min on ice. For the staining of intracellular CD24, viable cells were first fixed in the Cytofix/Cytoperm buffer followed by staining with PE-labelled anti-CD24 antibody and isotype control in Perm/Wash buffer. Cells were analysed on an LSII cytometer (Becton Dickinson). For cell cycle progression, the cell monolayer was harvested after treatment with EDTA-trypsin, washed with ice-cold PBS and fixed in ice-cold 70% ethanol overnight at −20 °C. After washing twice with PBS, the cells were incubated in RNase A-PBS (100 μg ml −1 ) at 37 °C for 30 min. DNA was labelled with propidium iodide (50 μg ml −1 ; BD Biosciences) and analysed with an LSII flow cytometer and CELLQuest software (Becton Dickinson). The percentage of cells in G0/G1, S and G2/M phases was evaluated by analysing 2 × 10 4 cells using the ModFit LT 3.0 program (Becton Dickinson). Immunohistochemistry Normal and prostate cancer frozen samples were partially thawed at room temperature and then immersed in 10% formalin for 12 h at 8 °C and embedded in paraffin. Antigens were retrieved by microwaving in retrieval buffer (Dako) for 12 min. The ABC detection system was used for immunostaining according to the manufacturer’s protocol (Vectastain Elite ABC). The primary antibodies were incubated with tissues overnight at 4 °C. This incubation was followed by the ABC detection system using biotinylated anti-mouse/rabbit/rat IgG. The slides were counterstained with haematoxylin and mounted in xylene mounting medium for examination. Proximity ligation assay We conducted proximity ligation assays using Duolink In Situ Red Starter Kit Mouse/Rabbit (Cat#: DUO92101, Sigma-Aldrich) according to the manufacturer’s protocol. Du145 cells stabilized with lentivirus expressing either control shRNA or CD24 shRNA were seeded in chamber slides (Nunc Lab-Tek) and fixed with 4% paraformaldehyde. Rabbit anti-NPM (Cat#: sc-6013R, Santa Cruz Biotechnology, 1:100) and mouse anti-p14ARF (Cat#: 2407, Cell Signaling, 1:100) were used as primary antibodies. In silico analysis of CD24 expression and TP53 status CD24 expression data (RNA Seq) and TP53 mutation status for low-grade glioma, glioblastoma and prostate adenocarcinoma were obtained from the Memorial Sloan Kettering Cancer Genomics Portal 74,75 ( http://www.cbioportal.org/public-portal ; last accessed on 25 April 2014). A function was implemented in the R software ( http://www.r-project.org ) to make the distribution diagrams that depict RNAseq values for CD24 and CD45 among samples with WT or mutant TP53. The samples from a given cancer cohort were divided into CD24 hi or CD24 lo subcohorts based on whether the RNAseq reads were above or below the mean of the cohort. The Pearson’s χ 2 test was used to evaluate the statistical significance in the frequencies of TP53 mutation in the CD24 hi and CD24 lo subcohorts. Statistics The log-rank test was used for survival analysis, Student’s t -test was used for pairwise comparison, whereas Pearson’s χ 2 test was used for multiple group comparisons. The analysis of variance trend test was used for gene dosage effect. Tumour growth rates were compared by Fisher’s Least Significant Difference test. Unless specific P -values are provided, those that reached statistical significance are given as follows: * P <0.05; ** P <0.01; *** P <0.001. How to cite this article: Wang, L. et al . Intracellular CD24 disrupts the ARF–NPM interaction and enables mutational and viral oncogene-mediated p53 inactivation. Nat. Commun. 6:5909 doi: 10.1038/ncomms6909 (2015).